Post-fusion structural changes and their roles in exocytosis and endocytosis of dense-core vesicles Vesicle fusion with the plasma membrane generates an Ω-shaped membrane profile. Its pore is thought to dilate until flattening (full-collapse), followed by classical endocytosis to retrieve vesicles. Alternatively, the pore may close (kiss-and-run), but the triggering mechanisms and its endocytic roles remain poorly understood. Here, using confocal and stimulated emission depletion microscopy imaging of dense-core vesicles, we find that fusion-generated Ω-profiles may enlarge or shrink while maintaining vesicular membrane proteins. Closure of fusion-generated Ω-profiles, which produces various sizes of vesicles, is the dominant mechanism mediating rapid and slow endocytosis within ~1–30 s. Strong calcium influx triggers dynamin-mediated closure. Weak calcium influx does not promote closure, but facilitates the merging of Ω-profiles with the plasma membrane via shrinking rather than full-collapse. These results establish a model, termed Ω-exo–endocytosis, in which the fusion-generated Ω-profile may shrink to merge with the plasma membrane, change in size or change in size then close in response to calcium, which is the main mechanism to retrieve dense-core vesicles. Exocytosis, a process that involves the fusion of a vesicle with the plasma membrane to release vesicular contents, is crucial for many biological events, including brain activities and endocrine functions [1] . To maintain exocytosis, fused vesicles are recycled via endocytosis. There are at least two exo–endocytosis modes. One involves vesicle full-collapse (FC) into the plasma membrane and spread of vesicular membrane proteins [2] , [3] , followed by classical endocytosis involving membrane invagination and fission to recycle vesicles [4] , [5] , [6] . The other mode, called kiss-and-run (KR) [7] , [8] , involves fusion pore opening and closure [4] , [5] , [6] . Although these two modes have been widely accepted, the presumed structural changes have not been observed in live cells at sub-diffraction-limited resolution. Here we used confocal and stimulated emission depletion microscopy (STED) [9] at ~230 nm and 90 nm resolution, respectively, to resolve these hypothesized structural changes in live chromaffin cells containing ~300 nm dense-core vesicles. Although decades of studies in chromaffin cells contribute to forming the current FC/KR theory [4] , [6] , [10] , [11] , the physiological role and the trigger mechanism of KR remain unresolved [4] , [10] . KR, which was first detected as capacitance flickers in ~0.2 s [12] , [13] , [14] , was proposed to underlie an entire cell’s endocytosis [15] . However, endocytosis recorded from whole-cell capacitance measurements (whole-cell endocytosis) lasts for ~20–30 s [15] . This long time course is difficult to be accounted for by KR as brief as ~0.2 s. A slower form of KR, termed cavicapture, has been revealed through imaging vesicular membrane proteins [15] . However, cavicapture is not considered the dominant mechanism mediating whole-cell endocytosis [15] . In brief, KR has not been established as the dominant endocytic mode in chromaffin cells. Neither has it been established in other cell types [4] , [5] , [6] . Two factors might contribute to this situation. First, to assess the contribution of KR to whole-cell endocytosis, it is best to reconstruct the overall endocytosis from individual KR for comparison with the simultaneously recorded whole-cell endocytosis. This comparison is labour intensive because KR is not trivial to record [13] , [15] . Second, the stimulation condition and the mechanism that predominantly triggers KR remain elusive [4] , [5] , [6] , [16] . KR is proposed to be triggered by low calcium [17] , [18] , [19] . Paradoxically, higher calcium influx speeds up whole-cell endocytosis in chromaffin cells [20] , [21] and other cell types [22] , [23] , [24] . In the present work, we develop an imaging technique with high spatial and temporal resolution to visualize structural changes of fusion-generated Ω-shaped membrane profile while simultaneously monitoring whole-cell endocytosis with capacitance measurements in chromaffin cells. We find that Ω-profile does not dilate as predicted by the FC model or simply close its pore as predicted by the KR model, but dynamically changes in seven modes. These results establish a model that redefines FC and KR fusion as part of a larger spectrum of structural changes, with varied triggers and physiological roles. We suggest to redefine KR as rapid or slow closure of Ω-shaped profile, during which this profile may change in size before closure, resulting in various sizes of vesicles. Pore closure is mediated by dynamin and triggered by large calcium influx. It is the predominant mechanism mediating whole-cell rapid and slow endocytosis lasting for ~1–30 s. It may also mediate bulk endocytosis, a form of endocytosis that generates large vesicles [5] , [6] . Low calcium influx facilitates shrinking of the fusion-generated Ω-shaped profile, leading to the merge of the fused vesicle with the plasma membrane. These results call for substantial modification of the classical FC and KR model. Imaging Ω-profile at the instant of fusion To label Ω-shaped membrane profiles and assess its structural changes, primary cultured bovine chromaffin cells were bathed with membrane-impermeable fluorescent dyes ( Fig. 1a ) [25] . With Alexa Fluor 647 (A647, 30 μM) in the bath, cells were voltage clamped while imaged confocally every 5–15 ms at the cell-bottom (applies if not mentioned otherwise, Fig. 1a ). A 1 s depolarization (depol 1s , from −80 mV to +10 mV, if not mentioned otherwise) induced a calcium current (ICa) of 309±34 pA (mean ±s.e.m., n =60), a capacitance jump (ΔCm) of 365±33 fF ( n =60) and 10.6±1.2 fluorescent A647 spots in ~70–160 μm 2 of the foot area of the cell ( n =60 cells, Fig. 1b ). This stimulation protocol was used because it consistently induces endocytosis ( Fig. 1b ) [15] , [26] . 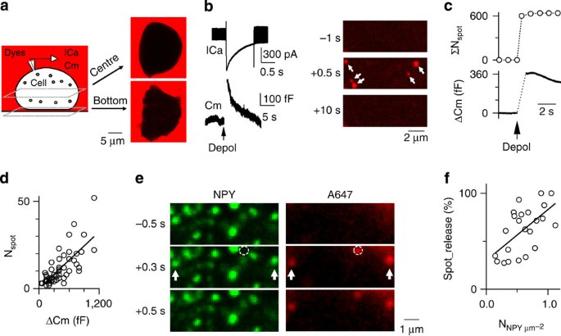Figure 1: Imaging granule fusion in chromaffin cells. (a) Left: Schematic drawing showing whole-cell recording of ICa and capacitance (Cm), and imaging at the cell-bottom or centre with a fluorescent dye (red) in the bath. Right: Confocal images at a real cell’s bottom (lower) or centre (upper) with A647 (30 μM) in the bath. The dark area at the cell-bottom represents a thin layer of A647 solution between the cell-bottom and the coverslip. (b) Left: Sampled ICa (upper) and Cm (lower) induced by depol1s(arrow). Right: A647 confocal/cell-bottom images at 1 s before, during (0.5 s) and 10 s after depol1s(same cell as from left). Arrows indicate A647 spots. (c) The accumulated number of A647 spots (ΣNspot, upper) plotted versus the time at which the spots occurred in 60 cells subjected to depol1s(arrow). The corresponding mean Cm change is also plotted (lower). (d) The A647 spot number (Nspot) plotted versus Cm from the same cell (n=60, each circle represents one cell). Data were fitted with a linear regression line (correlation coefficient: 0.71). (e) Concurrent imaging of NPY-EGFP (green) and A647 (red) at 0.5 s before (upper), and 0.3 s (middle) and 0.5 s (lower) during depol1s. Arrows indicate NPY-EGFP release (green spots disappeared at 0.5 s) coincident with A647 spots. Circles indicate an A647 spot without an overlapping NPY-EGFP spot. (f) The percentage of A647 spots that are co-localized with NPY-EGFP release (spot_release) plotted versus the number of NPY-EGFP granules per μm2at the cell-bottom (NNPYμm−2). Each circle represents one cell (n=23 cells; cells with>5 A647 spots were used). Figure 1: Imaging granule fusion in chromaffin cells. ( a ) Left: Schematic drawing showing whole-cell recording of ICa and capacitance (Cm), and imaging at the cell-bottom or centre with a fluorescent dye (red) in the bath. Right: Confocal images at a real cell’s bottom (lower) or centre (upper) with A647 (30 μM) in the bath. The dark area at the cell-bottom represents a thin layer of A647 solution between the cell-bottom and the coverslip. ( b ) Left: Sampled ICa (upper) and Cm (lower) induced by depol 1s (arrow). Right: A647 confocal/cell-bottom images at 1 s before, during (0.5 s) and 10 s after depol 1s (same cell as from left). Arrows indicate A647 spots. ( c ) The accumulated number of A647 spots (Σ N spot , upper) plotted versus the time at which the spots occurred in 60 cells subjected to depol 1s (arrow). The corresponding mean Cm change is also plotted (lower). ( d ) The A647 spot number ( N spot ) plotted versus Cm from the same cell ( n =60, each circle represents one cell). Data were fitted with a linear regression line (correlation coefficient: 0.71). ( e ) Concurrent imaging of NPY-EGFP (green) and A647 (red) at 0.5 s before (upper), and 0.3 s (middle) and 0.5 s (lower) during depol 1s . Arrows indicate NPY-EGFP release (green spots disappeared at 0.5 s) coincident with A647 spots. Circles indicate an A647 spot without an overlapping NPY-EGFP spot. ( f ) The percentage of A647 spots that are co-localized with NPY-EGFP release (spot_release) plotted versus the number of NPY-EGFP granules per μm 2 at the cell-bottom ( N NPY μm −2 ). Each circle represents one cell ( n =23 cells; cells with>5 A647 spots were used). Full size image Three sets of evidence suggest that A647 spots reflect vesicle fusion, owing to A647 diffusion from the bath to open vesicles. First, most spots occurred during and within 1 s after depolarization ( Fig. 1c , upper, 60 cells, 636 spots in total). This time course ( Fig. 1c , upper) was parallel to the immediate capacitance jump induced by depolarization, which reflects exocytosis ( Fig. 1c , lower). The spot number per cell was also proportional to the ΔCm ( Fig. 1d ). Second, analogous to calcium-triggered exocytosis, removing extracellular calcium abolished both spot occurrence and ΔCm ( n =10 cells, P <0.01, Supplementary Fig. 1 ). Third, in cells expressing neuropeptide Y-EGFP (NPY-EGFP, granule lumen cargo), 97% (=175/181) of the NPY-EGFP release events were accompanied with A647 spots ( Fig. 1e , arrows). The remaining 3% were likely too small or fast to be resolved. 58±5% of A647 spots ( n =350 spots, 23 cells) overlapped with NPY-EGFP-positive granules and their release ( Fig. 1e ). The percentage of overlap increased linearly towards 100% as the NPY-EGFP-positive granule density increased ( Fig. 1f ). Thus, A647 spots that did not overlap with NPY-EGFP-positive granules were due to fusion of NPY-EGFP-negative granules. Four sets of evidence suggest that the A647 spot at the onset reflects an Ω-profile at the fusion instant. First, under the confocal microscope, the full-width-half-maximum ( W H ) of NPY-EGFP-positive granule (475±13 nm, n =48 granules) was similar to the overlapping A647 spot’s W H at the onset (490±13 nm, n =48 spots, P =0.15, t -test; Fig. 2a ). STED imaging (~90 nm resolution) confirmed that the W H of NPY-EGFP-positive vesicle (332±5 nm, n =278 granules, 7 cells) was similar to the W H of spots (369±10 nm, n =101 spots, 31 cells) induced by depol 1s in different cells bathed with Alexa Fluor 488 (A488, 30–60 μM, Fig. 2b ). Note that A488 or EGFP, but not A647 can be used in our STED microscope. The spot W H measured with STED microscopy was close to electron microscopic measurements (~300 nm) [13] , supporting the idea that fused vesicles do not collapse. 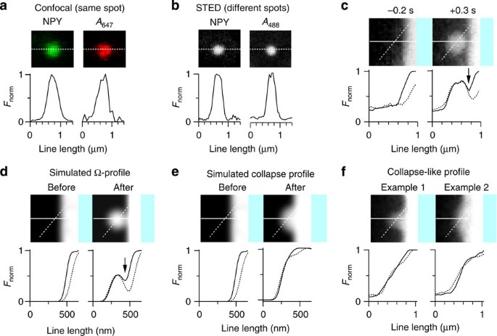Figure 2: Resolving the Ω-profile at the fusion instant. (a) Confocal images of a NPY-EGFP-positive granule before release and the A647 spot at the spot onset at the same location (upper). Normalized fluorescence intensity profiles (Fnorm) from dotted lines are also shown (lower, applies tob). (b) STED images (upper) of a NPY-EGFP granule and an A488 spot at the spot onset (from different cells). Line profiles are also plotted (lower). (c) STED/cell centre images at 0.2 s before (left) and 0.3 s (right) during depol1s(upper).Fnormare also shown for two lines across the spot centre, one perpendicular to the plasma membrane, the other 45° apart (applies tod–f). The arrow indicates the typical feature of the Ω-profile: a dip in the line profile that is wider and larger for the 45° line. Bright fluorescence in the right side of each image represents extracellular A488, whereas dim fluorescence in the left side of each image means the intracellular compartment with no A488 (applies to all plots at the STED per cell-centre setting). (d,e) Simulation showing side images and line profiles (solid and dotted) before (left) and after (right) the appearance of an Ω-profile (d, pore size: 50 nm, vesicle size: 300 nm) or a collapsed profile (e). The arrow in d indicates the typical feature of the Ω-profile: a dip in the line profile which is wider and larger for the 45° line. Images are taken fromSupplementary Figs 2f,g and 3c. Simulation methods are described inSupplementary Figs 2,3. (f) Two STED/cell-centre images and line profiles (left, right) that resemble the presumed collapsed profile. Images were obtained in resting conditions. Figure 2: Resolving the Ω-profile at the fusion instant. ( a ) Confocal images of a NPY-EGFP-positive granule before release and the A647 spot at the spot onset at the same location (upper). Normalized fluorescence intensity profiles ( F norm ) from dotted lines are also shown (lower, applies to b ). ( b ) STED images (upper) of a NPY-EGFP granule and an A488 spot at the spot onset (from different cells). Line profiles are also plotted (lower). ( c ) STED/cell centre images at 0.2 s before (left) and 0.3 s (right) during depol 1s (upper). F norm are also shown for two lines across the spot centre, one perpendicular to the plasma membrane, the other 45° apart (applies to d – f ). The arrow indicates the typical feature of the Ω-profile: a dip in the line profile that is wider and larger for the 45° line. Bright fluorescence in the right side of each image represents extracellular A488, whereas dim fluorescence in the left side of each image means the intracellular compartment with no A488 (applies to all plots at the STED per cell-centre setting). ( d , e ) Simulation showing side images and line profiles (solid and dotted) before (left) and after (right) the appearance of an Ω-profile ( d , pore size: 50 nm, vesicle size: 300 nm) or a collapsed profile ( e ). The arrow in d indicates the typical feature of the Ω-profile: a dip in the line profile which is wider and larger for the 45° line. Images are taken from Supplementary Figs 2f,g and 3c . Simulation methods are described in Supplementary Figs 2,3 . ( f ) Two STED/cell-centre images and line profiles (left, right) that resemble the presumed collapsed profile. Images were obtained in resting conditions. Full size image Second, to visualize these structures, we conducted STED imaging at the cell-centre (>2 μm above bottom), where the plasma membrane was approximately perpendicular to the coverslip ( Fig. 1a ). Depol 1s induced A488 spots only adjacent to the cell membrane ( Fig. 2c , n =45). These ‘side’ images showed Ω-like profiles with a pore beyond our resolution ( Fig. 2c ). To quantify the Ω-profile, we simulated an Ω-profile with a diameter of 300 nm and a pore <100 nm ( Fig. 2d , see Supplementary Fig. 2 for derivation). With a dye outside the cell membrane, line profiles through the simulated Ω-profile centre showed a dip right before reaching the membrane ( Fig. 2d , arrow). As expected for an Ω-profile, the dip for a 45° line was larger and wider than a horizontal line ( Fig. 2d ). These features were not observed in a simulated ‘FC’ profile with an opening that is the same or larger than the vesicle diameter ( Fig. 2e , Supplementary Fig. 3 ). The image and line features of the simulated Ω-profile were also observed in STED side images of A488 spots ( Fig. 2c , arrow), confirming that A488 spots were Ω-profiles. After depolarization, we did not observe spots that resembled the simulated collapse-like images and line features (see Methods for criteria of side imaging). However, we did observe some resting membrane curvatures ( Fig. 2f ) resembling the simulated ‘collapse’ image and line features ( Fig. 2e ). Thus, the lack of ‘collapse' profiles after depolarization was not due to limited spatial resolution. Third, the Ω-profile appeared at the spot onset (within 36 ms, our time resolution, 45 spots, see also Figs 3 , 4 , 5 ). This rapid appearance, together with the overlap between the spot appearance and NPY-EGFP release ( Fig. 1e,f ), suggests that the Ω-profile is due to fusion, but not slow, endocytic membrane invagination. 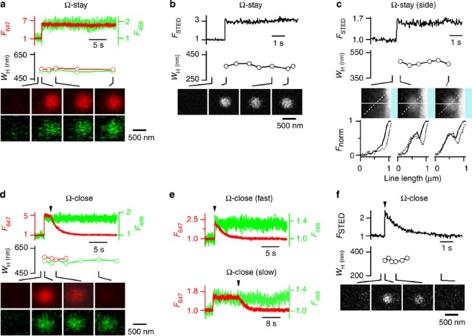Figure 3: Ω-stay and Ω-close fusion. (a–c), Ω-stay. (a)F647(red),F488(green),WHand sampled images (average of 4) at times indicated (lines) are plotted versus time for a spot at the confocalA647/A488 setting (cell-bottom).F647andF488were normalized to the mean value before spot appeared (applies to all plots ofF647,F488, andFSTED). Images were collected every 15 ms. (b)FSTED(STED fluorescence intensity),WH, and sampled images (average of 2) at times indicated are plotted versus time for a spot at the STED/cell-bottom setting (60 μM A488 in bath). Images were collected every 26 ms. (c)FSTED,WH, sampled images (average of 8, side images of the Ω-profile) and their line profiles (normalized to peak,Fnorm) are plotted versus time for a spot at the STED/cell-centre setting. Images were collected every 36 ms.WHwas measured from the profile of a vertical line (not shown, parallel to cell membrane) across the spot centre. Solid and dotted line profiles correspond to solid and dotted lines, respectively. The arrangements ina,bandcapply to all plots inFigs 3,4,5,6at confocal/A647/A488, STED/cell-bottom, and STED/cell-centre setting, respectively. (d–f) Ω-close at confocal/A647/A488 (d,e) and STED/cell-bottom setting (f). Arrows indicate pore closure (apply to ‘close’ fusion inFigs 3,4,5,6).Eshows two spots (upper, lower) with different pore closing time (WHand sampled images not shown). Figure 3: Ω-stay and Ω-close fusion. ( a – c ), Ω-stay. ( a ) F 647 (red), F 488 (green), W H and sampled images (average of 4) at times indicated (lines) are plotted versus time for a spot at the confocalA647/A488 setting (cell-bottom). F 647 and F 488 were normalized to the mean value before spot appeared (applies to all plots of F 647 , F 488 , and F STED ). Images were collected every 15 ms. ( b ) F STED (STED fluorescence intensity), W H , and sampled images (average of 2) at times indicated are plotted versus time for a spot at the STED/cell-bottom setting (60 μM A488 in bath). Images were collected every 26 ms. ( c ) F STED , W H , sampled images (average of 8, side images of the Ω-profile) and their line profiles (normalized to peak, F norm ) are plotted versus time for a spot at the STED/cell-centre setting. Images were collected every 36 ms. W H was measured from the profile of a vertical line (not shown, parallel to cell membrane) across the spot centre. Solid and dotted line profiles correspond to solid and dotted lines, respectively. The arrangements in a , b and c apply to all plots in Figs 3 , 4 , 5 , 6 at confocal/A647/A488, STED/cell-bottom, and STED/cell-centre setting, respectively. ( d – f ) Ω-close at confocal/A647/A488 ( d , e ) and STED/cell-bottom setting ( f ). Arrows indicate pore closure (apply to ‘close’ fusion in Figs 3 , 4 , 5 , 6 ). E shows two spots (upper, lower) with different pore closing time ( W H and sampled images not shown). 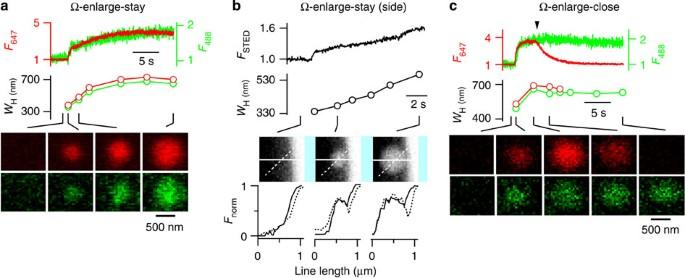Figure 4: Ω-enlarge-stay and Ω-enlarge-close. (a,b) Ω-enlarge-stay at confocal/A647/A488 (a) and STED/cell-centre setting (b). (c) Ω-enlarge-close at confocal/A647/A488 setting. Full size image Figure 4: Ω-enlarge-stay and Ω-enlarge-close. ( a , b ) Ω-enlarge-stay at confocal/A647/A488 ( a ) and STED/cell-centre setting ( b ). ( c ) Ω-enlarge-close at confocal/A647/A488 setting. 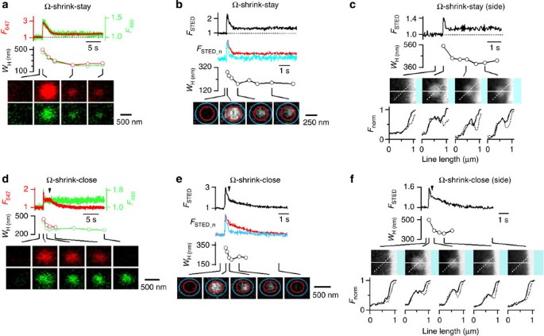Figure 5: Ω-shrink-stay and Ω-shrink-close. (a–c) Ω-shrink-stay at confocal/A647/A488 (a), STED/cell-bottom (b) and STED/cell-centre setting (c). Ina, the scale was set to see dim red images, but partly saturate the brightest red image. Inb,FSTED(peak normalized,FSTED_n) in the inner circle (red) and the outer ring (between red and blue circles, blue) are also plotted, showing faster decay of blue trace and thus the spot shrinkage. (c) Left two images, average of two single images; right two images, average of eight single images. (d–f) Ω-shrink-close at confocal/A647/A488 (d), STED/cell-bottom (e) and STED/cell-centre setting (f). Ine,FSTED_nin the inner circle (red) and the outer ring (between red and blue circles, blue) are also plotted to show spot shrinkage. (f) Left two images, average of two single images; right three images, average of eight single images. Full size image Figure 5: Ω-shrink-stay and Ω-shrink-close. ( a – c ) Ω-shrink-stay at confocal/A647/A488 ( a ), STED/cell-bottom ( b ) and STED/cell-centre setting ( c ). In a , the scale was set to see dim red images, but partly saturate the brightest red image. In b , F STED (peak normalized, F STED_n ) in the inner circle (red) and the outer ring (between red and blue circles, blue) are also plotted, showing faster decay of blue trace and thus the spot shrinkage. ( c ) Left two images, average of two single images; right two images, average of eight single images. ( d – f ) Ω-shrink-close at confocal/A647/A488 ( d ), STED/cell-bottom ( e ) and STED/cell-centre setting ( f ). In e , F STED_n in the inner circle (red) and the outer ring (between red and blue circles, blue) are also plotted to show spot shrinkage. ( f ) Left two images, average of two single images; right three images, average of eight single images. Full size image Fourth, some spots may close their pore without detectable structural changes (for example, Ω-close fusion, described later), confirming that the Ω-profile’s pore is too small to be resolved. Seven modes of Ω-profile change To determine how Ω-shaped membrane profiles change in size and pore opening or closing status, we performed confocal imaging (every 5–15 ms) at the cell-bottom with A647 and A488 in the bath being excited strongly and weakly, respectively (A647/A488 experiments, reasons explained later). We found that the structures may change in seven ways described below (636 spots, 60 cells), which reflect different size changes of the Ω-profile (no change, enlarge, shrink partially or completely) and the pore status (opened or closed). These patterns were confirmed with STED imaging at the cell-bottom (STED/cell-bottom, every 26 ms, strong excitation) and cell-centre (STED/cell-centre, every 36 ms, strong excitation). In 11% of the spots (73/636 spots) in confocal/A647/A488 experiments, A647 and A488 fluorescence intensity ( F 647 , F 488 ) peaked mostly rapidly (<100 ms) and stayed unchanged (<25%) for 30 s (the end of our image recording), during which A647 or A488 spot’s W H remained stable (A647: 485±8 nm at onset, 474±7 nm 30 s later, n =73 spots; P =0.56, t -test; Fig. 3a , Supplementary Movie 1 ). Similar results were confirmed with STED/cell-bottom imaging: W H was 380±35 nm at the onset, and was 400±40 nm 6–8 s later ( n =5; P =0.74; Fig. 3b ). STED data beyond ~8–10 s after stimulation were discarded, because the whole-cell configuration was often lost due to strong STED depletion laser. STED/cell-centre imaging showed an Ω-profile with a dip in line profiles, which remained stable for 6–8 s ( n =6, Fig. 3c ). This pattern is termed Ω-stay with an open pore. The evidence supporting an open pore is explained below. In 33% of the spots in A647/A488 experiments, F 647 and F 488 peaked simultaneously (<70 ms). Subsequently, F 647 remained unchanged for 0.3–30 s, then decayed monoexponentially to baseline with a τ of 2.9±0.1 s, whereas F 488 remained unchanged ( n =210 spots, Fig. 3d,e ; Supplementary Movie 2 ). The A647 or A488 spot’s W H also remained stable: A647 spot’s W H was 474±5 nm at the F 647 peak, and was 462±4 nm when F 647 decayed to 25±1% of the peak ( n =210, P =0.18, t -test; Fig. 3d,e ). STED/cell-bottom imaging confirmed this result: W H was 371±17 nm at the fluorescence ( F STED ) peak, and was 351±16 nm at 20–30% of F STED peak ( n =27, P =0.43, Fig. 3f ). This pattern, termed here as Ω-close, reflects Ω-profile pore closure resembling KR [7] , [8] , except that closing time can be long. The following two sets of evidence support this conclusion. First, when F 647 (strong excitation) but not F 488 decayed, removing A647 excitation halted F 647 decay, and resuming excitation recommenced F 647 decay ( n =11 spots, Supplementary Fig. 4a ). After F 647 decay, increasing A488 excitation increased F 488 , but followed by a monoexponential decay ( n =10 spots, Supplementary Fig. 4b ). Thus, strong excitation decreased F 647 (or F 488 ). However, strong excitation alone was insufficient to cause F 647 decay, because F 647 may remain stable (for example, Fig. 3a ) or decay at different onsets (for example, Fig. 3d,e ). Thus, F 647 decay must reflect pore closure, which prevents exchange of bleached dye (caused by strong excitation) with fluorescent dye in the bath. In contrast, a stable F 647 (Ω-stay) reflects an open pore ( Fig. 3a–c ). Second, as described later, endocytosis reconstructed from Ω-close and other ‘close’ modes matched whole-cell endocytosis. Moreover, block of whole-cell endocytosis by prolonging whole-cell dialysis or inhibition of dynamin abolished ‘close’ fusion. Thus, ‘close’ modes reflect endocytosis. In 8% of the spots in A647/A488 experiments, F 647 and F 488 increased in parallel in two phases, initially within ~300 ms and subsequently in~1–20 s ( Fig. 4a ). W H at the onset was 486±8 nm ( n =52), similar to Ω-stay (485±8 nm, n =73, P =0.78, t -test) or Ω-close (474±5 nm, n =210, P =0.14). It increased to 600±12 nm at the fluorescence peak ( n =52, P <0.001, Fig. 4a ). STED/cell-bottom imaging showed similar patterns: W H at the onset was 399±13 nm ( n =8), similar to that of Ω-stay (380±435 nm, n =5, P =0.60) or Ω-close (371±17 nm, n =27, P =0.42), but increased to 508±26 nm ( n =8) at the peak ( P <0.01). STED/cell-centre imaging revealed an Ω-profile (with a dip in line profiles) and its enlargement towards the cytosol ( n =6 spots, Fig. 4b , Supplementary Movie 3 ). This mode is termed Ω-enlarge-stay. The slow time course is not due to slow diffusion of the dye into the vesicle, but to the slow size increase, because the initial spot W H was similar to Ω-stay or Ω-close, and the dye diffuses to a granule in milliseconds [27] . About 2% of the spots in A647/A488 experiments showed initial changes similar to Ω-enlarge-stay, but followed by F 647 decay to baseline with a τ (2.8±0.2 s, n =15) similar to that of Ω-close while F 488 remained unchanged ( Fig. 4c ). This pattern reflected Ω-profile enlargement and closure, termed Ω-enlarge-close. In 13% of the spots in A647/A488 experiments, F 647 and F 488 peaked rapidly (<50 ms) and subsequently decreased in parallel by 50–89% with a τ of 273±41 ms ( n =84), then stayed unchanged for 30 s ( Fig. 5a ). W H at the onset was 505±8 nm, similar to that of Ω-stay, but decreased to 359±6 nm at the steady-state ( n =84, P <0.001, t -test, Fig. 5a ). STED/cell-bottom imaging confirmed the spot shrinkage: W H decreased from 379±26 to 237±18 nm ( n =22, P <0.01, t -test, Fig. 5b , Supplementary Movie 4 ), and the STED fluorescence intensity ( F STED ) in the spot’s outer ring decayed faster to a lower value near baseline than the spot’s centre ( n =22, for example, Fig. 5b ). Consistently, STED/cell-centre imaging showed that the Ω-profile (with a dip in line profiles) shrank towards the plasma membrane without vesicle budding off, then maintained the Ω-profile ( n =12 spots, Fig. 5c ), termed Ω-shrink-stay. In 14% of the spots in A647/A488 experiments, F 647 and F 488 showed initial patterns similar to Ω-shrink-stay, except that after a variable delay (0.3–30s) in the ‘stay’ phase, F 647 decayed to baseline with a τ (2.8±0.1 s, n =87) similar to that of Ω-close while F 488 remained unchanged ( Fig. 5d ). The spot W H was 509±7 nm at the onset, decreased to 418±5 nm ( n =87, P <0.001, t -test) at the temporary ‘stay’ phase, then remained unchanged as F 647 decayed (409±6 nm at ~30% of the ‘stay’ amplitude, n =87, P =0.51, t -test, Fig. 5d ). STED/cell-bottom imaging showed similar pattern: W H decreased from 356±18 nm at the onset to 244±12 nm ( n =20, P <0.001, t -test) at the temporary ‘stay’ phase, then remained stable as F STED decayed to baseline (254±13 nm at ~30% of amplitude at the transition phase, n =20, P =0.47, t -test; Fig. 5e ). F STED in the spot’s outer ring decayed faster to a lower value than the spot’s centre in the initial shrinking phase, indicating Ω-profile shrinkage ( n =20, for example, Fig. 5e ). Consistently, STED/cell-centre imaging showed that the Ω-profile (and the dip in line profiles) initially shrank towards the plasma membrane, then its size stayed unchanged while F STED decayed to baseline ( n =13 spots, Fig. 5f ). These results reflected the Ω-profile shrinkage and closure, termed Ω-shrink-close. In 18% of the spots in A647/A488 experiments, F 647 and F 488 peaked rapidly (<50 ms), then decreased in parallel to baseline with a τ (1.09±0.11 s, n =115, Fig. 6a,b ) faster than the dye bleaching τ during Ω-close (2.9±0.1 s, n =210, P <0.001, t -test). The decay τ was mostly less than 1.5 s, and sometimes only 15–50 ms ( Fig. 6b ). The W H decreased from 504±12 nm at the onset to 365±10 nm ( n =115) at 23±1% of the peak F 647 (for example, Fig. 6a ), beyond which W H was too dim to measure. STED/cell-bottom imaging confirmed this pattern: W H decreased from 362±33 nm at the onset to 225±27 nm at 16±2% of the F STED peak ( n =19, P <0.01, t -test; Fig. 6c , Supplementary Movie 5 ). F STED in the spot’s outer ring decayed faster than the centre ( n =19, Fig. 6c ), confirming Ω-profile shrinkage. STED/cell-centre imaging showed shrinkage of the Ω-profile (and the dip in line profile) without vesicle budding off ( n =8, Fig. 6d , Supplementary Movie 6 ), termed Ω-shrink. 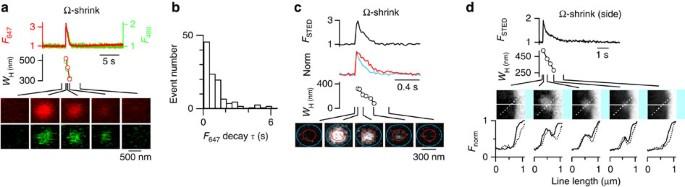Figure 6: Ω-shrink fusion. (a) Ω-shrink at confocal/A647/A488 setting. (b)Distribution of theF647decayτduring Ω-shrink fusion at confocal/A647/A488 setting (115 spots, 60 cells, data binned every 0.5 s). (c,d) Ω-shrink at STED/cell-bottom (c) and STED/cell-centre setting (d). Inc,FSTED_nin the inner circle (red) and the outer ring (blue) are also plotted to show spot shrinkage. (d) Left two images, average of two single images; right three images, average of eight single images. Figure 6: Ω-shrink fusion. ( a ) Ω-shrink at confocal/A647/A488 setting. ( b )Distribution of the F 647 decay τ during Ω-shrink fusion at confocal/A647/A488 setting (115 spots, 60 cells, data binned every 0.5 s). ( c , d ) Ω-shrink at STED/cell-bottom ( c ) and STED/cell-centre setting ( d ). In c , F STED_n in the inner circle (red) and the outer ring (blue) are also plotted to show spot shrinkage. ( d ) Left two images, average of two single images; right three images, average of eight single images. Full size image In summary, we described seven ways in which an Ω-shaped membrane profile can change, including three close modes (Ω-close, Ω-enlarge-close, Ω-shrink-close), three stay modes (Ω-stay, Ω-enlarge-stay, Ω-shrink-stay) and Ω-shrink ( Fig. 7a ). Since we limited imaging to 30 s, pore closure for stay modes beyond 30 s is possible. In addition, we observed occasional events not following these typical patterns. Atypical changes included pore closure and reopening, reflected as F 647 bleaching (pore closure) and sudden increase to the original level (pore reopening) while F 488 remained unchanged; Ω-stay followed by Ω-shrink or Ω-shrink-stay, reflected as stable F 647 value followed by parallel decrease of F 647 and F 488 ; and Ω-enlarge-stay followed by Ω-shrink-stay, reflected as parallel increase and then decrease of both F 647 and F 488 . These events reflect the continuous nature and flexibility of post-fusion structural changes. 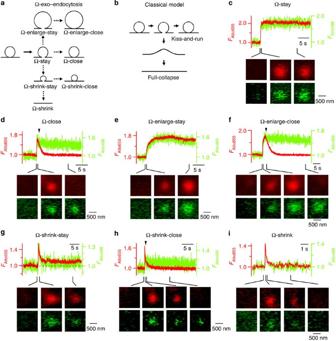Figure 7: Seven fusion modes confirmed by imaging with Atto 655 and Atto 488. (a,b) Schematic drawings of our model called Ω-exo–endocytosis (a, seven modes) and the classical FC and KR model (b). Dotted arrows mean that the transition may or may not take place. (c) Atto 655 fluorescence intensity (FAtto655, red), Atto 488 fluorescence intensity (FAtto488, green) and sampled images (average of 5–10 frames) at times indicated (lines) are plotted versus time for a spot undergoing Ω-stay fusion.FAtto655andFAtto488were normalized to the mean value before spot appeared. Images were collected every 17–34 ms at the confocal cell-bottom setting with Atto 655 (strong excitation) and Atto 488 (weak excitation) in the bath. (d–i) Similar toc, but for spots undergoing Ω-close (d), Ω-enlarge-stay (e), Ω-enlarge-close (f), Ω-shrink-stay (g), Ω-shrink-close (h) and Ω-shrink (i). Figure 7: Seven fusion modes confirmed by imaging with Atto 655 and Atto 488. ( a , b ) Schematic drawings of our model called Ω-exo–endocytosis ( a , seven modes) and the classical FC and KR model ( b ). Dotted arrows mean that the transition may or may not take place. ( c ) Atto 655 fluorescence intensity ( F Atto655 , red), Atto 488 fluorescence intensity ( F Atto488 , green) and sampled images (average of 5–10 frames) at times indicated (lines) are plotted versus time for a spot undergoing Ω-stay fusion. F Atto655 and F Atto488 were normalized to the mean value before spot appeared. Images were collected every 17–34 ms at the confocal cell-bottom setting with Atto 655 (strong excitation) and Atto 488 (weak excitation) in the bath. ( d – i ) Similar to c , but for spots undergoing Ω-close ( d ), Ω-enlarge-stay ( e ), Ω-enlarge-close ( f ), Ω-shrink-stay ( g ), Ω-shrink-close ( h ) and Ω-shrink ( i ). Full size image No FC fusion We did not observe FC fusion ( Fig. 7b ). The predicted structural change of FC would be spot enlargement while dimming at the cell-bottom, and the collapse of the Ω-profile ( Fig. 2e,f ) at side images. Neither of these structural changes was observed after stimulation. Thus, FC fusion was inexistent or rare. This suggestion was not due to limit in time resolution, because we imaged every 5–15 ms, which detected nearly all NPY-EGFP releasing granules (for example, Fig. 1e ). It was also not due to the stimulus we used (depol 1s ), because FC fusion was absent with two other stimuli: a 2-ms depolarization train at 5–15 Hz for 30 s that mimicked an action potential train (48 spots, 5 cells), and high potassium application (50 mM, 53 spots, 4 cells). Spot size changes are not caused by movement The spot enlargement or shrinking we observed was not due to focal plane changes, because while some spots enlarged or shrank, pre-existing fluorescent structures 1–2 μm away did not change ( Supplementary Fig. 5a–c ). Could it be due to localized (<1–2 μm) membrane movement that pushes the Ω-shaped membrane profile into the cytosol in the z axis? Four sets of evidence exclude this possibility. First, the fluorescence within ~0.5–1 μm surrounding the spot remained unchanged at the STED cell-bottom setting ( n =101 spots, for example, Supplementary Fig. 6 ), indicating no movement surrounding the spot. Similar results were observed using FM4–64 to label membrane ( Supplementary Fig. 7a ) [28] and Atto 488 to identify fusion modes ( n =75 spots, 6 cells, Supplementary Fig. 7b–d ). Second, at the cell-centre setting where the movement to the cytosol could be resolved at the microscopic x/y plane (illustrated in Supplementary Fig. 8c–e ), we did not observe any such movements ( n =45 spots; for example, Supplementary Fig. 8f–j ). Third, at a z resolution of ~100–150 nm total internal reflection fluorescence microscopy (TIRF, cell-bottom setting, 30 μM Alexa 555 in bath) showed that after depol 1s the spot size may shrink completely (Ω-shrink, 33 out of 178 spots, Supplementary Fig. 9a ), shrink partially (including Ω-shrink-stay and Ω-shrink-close; 33/178 spots, Supplementary Fig. 9b ), enlarge (including Ω-enlarge-stay and Ω-enlarge-close; 17/178 spots, Supplementary Fig. 9c ), or remain unchanged (including Ω-stay and Ω-close; 95/178 spots, Supplementary Fig. 9d ). This result excludes movements to the cytosol of ~350 nm or larger (the confocal z resolution is ± ~350 nm) as the cause for spot size changes. Fourth, to monitor such movements at STED cell-bottom setting (A488 in bath), we switched the focal plane every 70 ms between the cell-bottom (control) and a focal plane that was 300 nm above (upper). Spots induced by depol 1s were brighter and focused at the control focal plane, but dimmer and out of focus at the upper focal plane (131 spots). When spots dimmed and shrank completely (28 spots, Supplementary Fig. 10a ) or partially (40 spots, Supplementary Fig. 10b ) at the control plane, F STED at the upper plane also decreased, but slightly faster ( Supplementary Fig. 10a,b ). Thus, spot shrinking at the control plane is not due to an upward movement towards the cytosol. Similarly, all spots (21 spots) that became brighter and larger at the control plane were also brighter at the upper plane ( Supplementary Fig. 10c ). In conclusion, the spot size change we observed is not due to movement to the cytosol, but to actual structural changes. Seven modes observed with other image settings The seven modes were not only observed with the A647/A488 setting, but also with other settings, which validates our observations. When we used only one dye (A647) and excited it weakly, the spot size could remain the same ( n =42 spots), increase ( n =7 spots), or decrease (to some extent or till undetectable, n =23 spots; Supplementary Fig. 11 ; 7 cells), indicating that the spot size changes were not due to photo-toxicity caused by strong excitation. When we excited A488 strongly, but A647 weakly, depol 1s induced 62 spots (9 cells) showing six modes (Ω-stay, 9 spots; Ω-close, 12 spots; Ω-enlarge-stay, 6 spots; Ω-enlarge-close, 0 spots; Ω-shrink-stay, 9 spots; Ω-shrink-close, 15 spots; Ω-shrink, 11 spots; Supplementary Fig. 12 ). When we replaced A647 and A488 with Atto 655 (strong excitation/confocal) and Atto 488 (weak excitation/confocal), depol 1s induced 143 spots (7 cells) showing seven modes (Ω-stay, 8 spots; Ω-close, 45 spots; Ω-enlarge-stay, 7 spots; Ω-enlarge-close, 3 spots; Ω-shrink-stay, 19 spots; Ω-shrink-close, 31 spots; Ω-shrink, 30 spots; Fig. 7c–i ). With these settings, the percentage of each mode (obtained from smaller data sets) was roughly similar to those obtained with A647/A488 setting. Three close modes mediate rapid and slow endocytosis Three sets of evidence in A647/A488 experiments suggest that close fusion (Ω-close, Ω-shrink-close, Ω-enlarge-close) mediates whole-cell rapid (a few seconds) and slow (tens of seconds) endocytosis. First, if we assigned an upstep at every spot’s onset and a downstep at pore closing time ( F 647 decay onset) with an amplitude correction for Ω-shrink-close and Ω-enlarge-close ( Fig. 8a , see Methods), the up and downstep interval in close events ranged from 0.3–30 s ( n =312; Fig. 8b ), covering both rapid and slow endocytic time frame. 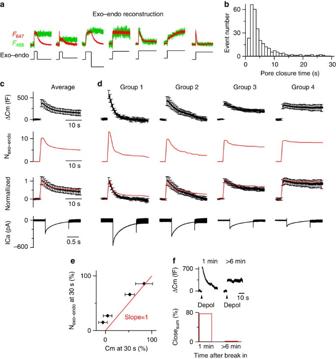Figure 8: Close modes mediate rapid and slow endocytosis of the cell. (a) Examples showing net exo– and endocytosis (lower: exo–endo, see also Methods) reconstructed from fluorescence changes (upper:F647,F488) during Ω-close, Ω-shrink-close, Ω-enlarge-close, Ω-stay, Ω-shrink-stay, Ω-enlarge-stay and Ω-shrink fusion (left to right). (b) Pore closure time (from open to close, not from stimulation time to closure) distribution for three ‘close’ modes (312 spots). (c) The mean Cm (±s.e.m., every 1 s, baseline subtracted, upper),Nexo–endoper cell (middle upper) and ICa (lower) induced by depol1s(to +10 mV). Cm (black) andNexo–endo(red) traces are also normalized and superimposed for comparison (middle lower). Data were from 636 spots in 60 cells. (d) Similar toc, except that data incwere divided into four groups based on Cm decay: (1) decay to baseline in 15 s (165 spots, 11 cells), (2) decay by >80% in 30 s except group 1 (101 spots, 10 cells), (3) decay by 30–80% in 30 s (173 spots, 18 cells) and (4) decay by <30% in 30 s (197 spots, 21 cells). (e) The percentage ofNexo–endoat 30 s after depol1s(compared with the peakNexo–endo) plotted versus the corresponding undecayed Cm percentage at 30 s after stimulation from four groups described ind(left to right, group 1–4). A line (red) with a slope of 1 is also plotted. Error bars are s.e.m. The spot number and cell number are described ind. (f) The mean Cm change (upper, ΔCm) and the percentage of close fusion (Closesum, lower, including Ω-close, Ω-shrink-close and Ω-enlarge-close) induced by depol1swithin 1 min (left, 53/68 spots are ‘close’ fusion) and >6 min (right, 1/31 spots is close fusion) after whole-cell break-in from the same cell (n=4 cells). Figure 8: Close modes mediate rapid and slow endocytosis of the cell. ( a ) Examples showing net exo– and endocytosis (lower: exo–endo, see also Methods) reconstructed from fluorescence changes (upper: F 647 , F 488 ) during Ω-close, Ω-shrink-close, Ω-enlarge-close, Ω-stay, Ω-shrink-stay, Ω-enlarge-stay and Ω-shrink fusion (left to right). ( b ) Pore closure time (from open to close, not from stimulation time to closure) distribution for three ‘close’ modes (312 spots). ( c ) The mean Cm (±s.e.m., every 1 s, baseline subtracted, upper), N exo–endo per cell (middle upper) and ICa (lower) induced by depol 1s (to +10 mV). Cm (black) and N exo–endo (red) traces are also normalized and superimposed for comparison (middle lower). Data were from 636 spots in 60 cells. ( d ) Similar to c , except that data in c were divided into four groups based on Cm decay: (1) decay to baseline in 15 s (165 spots, 11 cells), (2) decay by >80% in 30 s except group 1 (101 spots, 10 cells), (3) decay by 30–80% in 30 s (173 spots, 18 cells) and (4) decay by <30% in 30 s (197 spots, 21 cells). ( e ) The percentage of N exo–endo at 30 s after depol 1s (compared with the peak N exo–endo ) plotted versus the corresponding undecayed Cm percentage at 30 s after stimulation from four groups described in d (left to right, group 1–4). A line (red) with a slope of 1 is also plotted. Error bars are s.e.m. The spot number and cell number are described in d . ( f ) The mean Cm change (upper, ΔCm) and the percentage of close fusion (Close sum , lower, including Ω-close, Ω-shrink-close and Ω-enlarge-close) induced by depol 1s within 1 min (left, 53/68 spots are ‘close’ fusion) and >6 min (right, 1/31 spots is close fusion) after whole-cell break-in from the same cell ( n =4 cells). Full size image Second, summation of the up and downsteps from all spots (636 spots) yielded reconstructed net exo– and endocytosis ( N exo–endo , Fig. 8c , red), which matched approximately the corresponding whole-cell endocytosis ( Fig. 8c , black, 60 cells) in both time course and amplitude. The match was also observed when we divided cells into four groups based on capacitance decay: decay to baseline within 15 s (group 1), decay by >80% in 30 s (group 2, not including group 1), decay by 30–80% in 30 s (group 3) and decay by <30% in 30 s (group 4, Fig. 8d ). N exo–endo and capacitance decayed rapidly with a τ of 2.8 s and 3.9 s, respectively, in group 1; but decayed slowly with a τ of 8.1 and 13.8 s, respectively, in group 2. In groups 3–4, N exo–endo and capacitance changes were similar and did not return to baseline. The fraction that did not decay for N exo–endo and capacitance was similar in all groups ( Fig. 8e ). These results suggest that close modes mediate most whole-cell rapid and slow endocytosis. Third, since prolonged whole-cell dialysis blocks endocytosis [21] , [29] , we used this feature to determine whether close modes cause whole-cell endocytosis. In 4 cells, depol 1s induced whole-cell endocytosis and 78% (53/68 spots) close fusion within 1 min after break-in, but induced no whole-cell endocytosis, and only 3% close fusion (1/31 spots, Fig. 8f , n=4 cells) 6 min later, suggesting that close modes cause whole-cell endocytosis. Calcium influx determines fusion modes From group 4 to 1, ICa increased from 175±25 pA ( n =21 cells) to 576±61 pA ( n =11 cells, Fig. 8d ), close events (three close modes) increased and became dominant, whereas the stay events (three stay modes) and Ω-shrink decreased ( Fig. 9a ). The correlation between ICa and close fusion ( Fig. 9a , red), between ICa and stay fusion ( Fig. 9a blue), and between ICa and Ω-shrink ( Fig. 9a , black) are causal, because in cells showing large ICa (>450 pA during <10 ms depolarization to +10 mV), when we reduced ICa using a 1-s depolarization to +50 mV (102±8 pA, n =12 cells, Fig. 9b ), close events were nearly fully blocked (3.1%), whereas stay events and Ω-shrink increased ( Fig. 9c , open symbols, 12 cells, 64 spots). Thus, large ICa triggered close modes, whereas low ICa promoted stay modes and Ω-shrink. 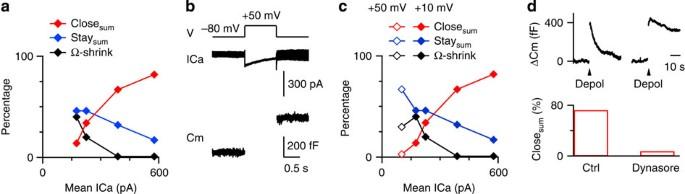Figure 9: Strong calcium influx triggers dynamin-dependent close fusion modes and low calcium promotes stay modes and Ω-shrink. (a) The percentage of Closesum(including all three close modes), Staysum(including three stay modes) and Ω-shrink plotted versus the mean ICa in four groups described inFig. 8d(stimulation: depol1sto +10 mV). The percentage was calculated within each group. (b) Sample ICa and Cm induced by a 1 s depolarization to +50 mV. This cell showed an ICa of ~500 pA during a 10 ms depolarization to +10 mV (not shown). (c) Re-plottinga(solid symbols), but including data similar to those shown inb(open symbols), where 1 s depolarization to +50 mV induced the smallest ICa as compared with the mean ICa induced by depol1sto +10 mV in groups 1–4. (d) The mean Cm change (upper, ΔCm) and the percentage of close fusion (Closesum, lower, including Ω-close, Ω-shrink-close and Ω-enlarge-close) induced by depol1sin control (10 cells, 66 spots, left) and in cells bathed with 80 μM dynasore (14 cells, 63 spots, right). In both groups, cells with an ICa>350 pA were selected for analysis. Figure 9: Strong calcium influx triggers dynamin-dependent close fusion modes and low calcium promotes stay modes and Ω-shrink. ( a ) The percentage of Close sum (including all three close modes), Stay sum (including three stay modes) and Ω-shrink plotted versus the mean ICa in four groups described in Fig. 8d (stimulation: depol 1s to +10 mV). The percentage was calculated within each group. ( b ) Sample ICa and Cm induced by a 1 s depolarization to +50 mV. This cell showed an ICa of ~500 pA during a 10 ms depolarization to +10 mV (not shown). ( c ) Re-plotting a (solid symbols), but including data similar to those shown in b (open symbols), where 1 s depolarization to +50 mV induced the smallest ICa as compared with the mean ICa induced by depol 1s to +10 mV in groups 1–4. ( d ) The mean Cm change (upper, ΔCm) and the percentage of close fusion (Close sum , lower, including Ω-close, Ω-shrink-close and Ω-enlarge-close) induced by depol 1s in control (10 cells, 66 spots, left) and in cells bathed with 80 μM dynasore (14 cells, 63 spots, right). In both groups, cells with an ICa>350 pA were selected for analysis. Full size image Dynamin mediates fusion pore closure In control cells with an Ica >350 pA (mean: 499±54 pA, n =10 cells), depol 1s induced whole-cell endocytosis and 73% (48/66 spots) of close fusion ( Fig. 9d ). With the dynamin inhibitor dynasore (80 μM, 20–30 min) in the bath in cells with an ICa >350 pA (mean: 515±41 pA, n =14 cells), depol 1s induced nearly no whole-cell endocytosis (~10–30% at 30 s after depol 1s , Fig. 9d ) and only 8% (5/63 spots) close fusion ( Fig. 9d ). Similarly, including in the pipette solution the dynamin inhibitory peptide (QVPSRPNRAP, 20 μM; Tocris) [30] , which inhibits dynamin interaction with amphiphysin, largely blocked whole-cell endocytosis and reduced close fusion to 9% (4/45 spots) in cells with an ICa>350 pA (585±73 pA, n =6). These results suggest that dynamin mediates fusion pore closure, which in turn mediates whole-cell rapid and slow endocytosis. Ω-profile retains vesicular membrane protein To determine whether the Ω-shaped membrane profile, which was observed in all seven modes, holds vesicular membrane proteins from diffusion, we imaged cells expressing a vesicular membrane protein VAMP2 tagged with EGFP (VAMP2-EGFP, weak excitation). A647 (bath, strong excitation) was included for identifying fusion modes (see Methods and Supplementary Fig. 13 ). Depol 1s induced 66 A647 spots (14 cells) that coincided with VAMP2-EGFP spots. VAMP2-EGFP fluorescence ( F VAMP2 ) increased at A647 spot onset owing to the pH increase upon fusion ( Fig. 10 ) [31] . 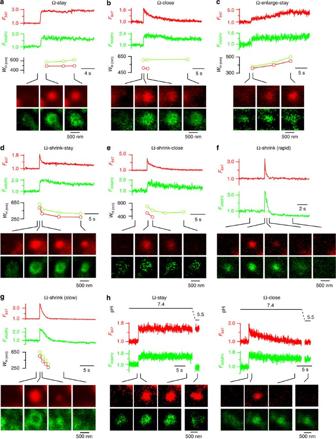Figure 10: Ω-profile retains vesicle membrane protein VAMP2. (a–g)F647(red),FVAMP2(green),WHof A647 (red) and VAMP2-EGFP (green) spot, and sampled A647 (red) and VAMP2-EGFP (green) images (at times indicated with lines) for spots undergoing Ω-stay (a), Ω-close (b), Ω-enlarge-stay (c), Ω-shrink-stay (d), Ω-shrink-close (e) and Ω-shrink (f: rapid shrinking, diffusion cloud;g: slow shrinking, size reduction observed). Cells were expressed with VAMP2-EGFP and stimulated by depol1swith A647 in the bath.WHis not measured inf, because VAMP2-EGFP rapidly diffused into a cloud, which did not reflect the Ω-shaped membrane profile size. VAMP2-EGFP spots appeared slightly (~50–100 nm inWH) larger than corresponding A647 spots (for example,Fig. 10a,b), because VAMP2-EGFP was located at the membrane, whereas A647 was inside the Ω-shaped structure. (h) TheF647andFVAMP2changes in response to a bath pH change from 7.4 to 5.5 (upper) for spots undergoing Ω-stay (left) and Ω-close (right). Figure 10: Ω-profile retains vesicle membrane protein VAMP2. ( a – g ) F 647 (red), F VAMP2 (green), W H of A647 (red) and VAMP2-EGFP (green) spot, and sampled A647 (red) and VAMP2-EGFP (green) images (at times indicated with lines) for spots undergoing Ω-stay ( a ), Ω-close ( b ), Ω-enlarge-stay ( c ), Ω-shrink-stay ( d ), Ω-shrink-close ( e ) and Ω-shrink ( f : rapid shrinking, diffusion cloud; g : slow shrinking, size reduction observed). Cells were expressed with VAMP2-EGFP and stimulated by depol 1s with A647 in the bath. W H is not measured in f , because VAMP2-EGFP rapidly diffused into a cloud, which did not reflect the Ω-shaped membrane profile size. VAMP2-EGFP spots appeared slightly (~50–100 nm in W H ) larger than corresponding A647 spots (for example, Fig. 10a,b ), because VAMP2-EGFP was located at the membrane, whereas A647 was inside the Ω-shaped structure. ( h ) The F 647 and F VAMP2 changes in response to a bath pH change from 7.4 to 5.5 (upper) for spots undergoing Ω-stay (left) and Ω-close (right). Full size image During Ω-stay, F VAMP2 and spot size remained stable ( n =12 spots, Fig. 10a ). During Ω-close, spot size remained stable ( n =13 spots, Fig. 10b ). Pore closure lead to F 647 decay, whereas F VAMP2 decreased partially in 30 s ( n =13 spots, Fig. 10b ), consistent with cavicapture that takes 100 s or longer for re-acidification [15] , [31] . During Ω-enlarge-stay, F VAMP2 remained stable, whereas VAMP2-EGFP spot size increased ( n =5, Fig. 10c ). During Ω-shrink-stay, F 647 decrease (to 20±2%, n =9) in the shrink phase was not accompanied by parallel F VAMP2 decrease, but a delayed and smaller F VAMP2 decrease (to 67±7%, n =9, for example, Fig. 10d ). However, VAMP2-EGFP spot W H decreased in parallel with A647 spot W H (for example, Fig. 10d , n =9), suggesting that the Ω-shaped membrane prevents or slows down diffusion of vesicular membrane proteins. For Ω-shrink-close, A647 and VAMP2-EGFP spot size reduced in parallel (for example, Fig. 10e , n =5). F VAMP2 did not decay during the shrink phase just like Ω-shrink-stay, but decayed with a delay slowly ( n =5, Fig. 10e ), likely due to slow re-acidification [15] , [31] . During Ω-shrink, F VAMP2 decreased to baseline ( n =22). If shrinking was rapid, a VAMP2-EGFP diffusion cloud was observed ( Fig. 10f ). If shrinking was slow, VAMP2-EGFP spot size reduced in parallel with the A647 spot size ( Fig. 10g ). F VAMP2 reduction significantly lagged behind F 647 reduction, reminiscent of the delay observed in Ω-shrink-stay and Ω-shrink-close ( Fig. 10d,e ). Thus, in all seven modes, Ω-shaped membrane profiles may prevent or slow down diffusion of vesicular membrane proteins. At ~20 s after the spot appeared, reducing the bath pH to 5.5 by applying MES solution decreased the pH-sensitive F VAMP2 (ref. 31 ) to baseline for stay events (including Ω-stay, Ω-enlarge-stay and Ω-shrink-stay, n =9 spots, Fig. 10h , left), but not for close events (including Ω-close and Ω-shrink-close, n =8 spots, Fig. 10 , right), confirming the pore open or close status, as determined by A647 imaging. We establish a new exo–endocytosis model, termed Ω-exo–endocytosis ( Fig. 7a ), where the Ω-profile fuison does not dilate, but changes in seven patterns through size transformation and fusion pore closure. This model is fundamentally different from the classical FC/KR model. FC is redefined as Ω-shrink, which merges fused vesicles with the plasma membrane by shrinking, but not dilating the Ω-shaped membrane profile. KR is redefined as close fusion, including Ω-close, Ω-shrink-close and Ω-enlarge-close, which may generate different-sized vesicles. Close fusion is triggered by strong calcium influx and requires dynamin to close the pore. Close fusion is the dominant mechanism mediating whole-cell rapid and slow endocytosis. It may also regulate vesicle size by shrinking or enlarging the Ω-shaped membrane profile before fusion pore closure. Consequently, the enlargement (Ω-enlarge-close) may mediate bulk endocytosis, a form of endocytosis defined as formation of large vesicles from the plasma membrane [5] , [6] . While strong calcium influx triggers close fusion, weak calcium influx facilitates stay fusion (Ω-stay, Ω-shrink-stay, Ω-enlarge-stay) and Ω-shrink. Unlike the irreversible FC model, transition between the different modes in the Ω-exo–endocytosis model is flexible ( Fig. 7a ). Finally, most vesicular membrane proteins are maintained in the Ω-shaped membrane during various modes of fusion by a mechanism that needs further investigation. Our model may account for most observations previously interpreted with FC/KR model. For example, Ω-shrink not only accounts for the merging of fused vesicles with the plasma membrane previously attributed to FC, but also allows for the flexibility to close the fusion pore anytime during shrinking ( Fig. 7a ). The pore of Ω-shrink fusion is much larger than 4 nm, because Ω-shrink released the ~4 nm NPY-EGFP [32] rapidly with a τ of 33±4 ms ( n =49 spots, for example, Fig. 1e ). Ω-shrink with a large pore may explain all live-cell data previously interpreted as FC, such as rapid content release, fusion pore conductance increase above a detection limit (corresponds to ~3–5 nm pore), and disappearance of fusion-generated vesicular images in endocrine cells and neurons [13] , [15] , [25] , [27] , [31] , [33] , [34] , [35] , [36] , [37] . Could Ω-shrink replace FC at synapses? FC was first suggested by Heuser and Reese [2] based on freeze-fracture electron microscopic observation that there are more large openings (diameter: 60–120 nm) at 50 ms than at 3–5 ms after stimulation at neuromuscular junctions [38] . It predicts that as pore dilates, large openings become dominant. However, large openings are not dominant at any time measured [2] . Using similar techniques and preparation, Ceccarelli et al. [7] questioned whether FC exists [39] , [40] . A recent study shows a widened neck of an Ω-profile consistent with the FC model [41] . However, FC has not been observed in live cells. An increased surface area [42] and release of ~15 nm quantum dot [43] at live retinal and hippocampal nerve terminals support FC, but can also be interpreted with Ω-shrink that has a large pore. Further work is needed to confirm Ω-shrink fusion in live synapses. By comparing endocytosis reconstructed from 636 fusion events with concurrently measured whole-cell endocytosis, we found that fusion pore closure during close fusion mediates most slow endocytosis within 30 s after stimulation ( Fig. 8c , d , group 2–4). We cannot exclude classical endocytosis beyond 30 s, although closure of stay fusion may also contribute to whole-cell endocytosis. Our finding challenges the traditional view that slow endocytosis is mediated by classical endocytosis. Can close fusion contribute to slow endocytosis at synapses? Inhibition of slow endocytosis by blocking clathrin-dependent endocytosis [5] and the existence of a readily retrievable pool [44] , [45] , [46] argue against this possibility. However, it remains unclear whether close fusion is clathrin-dependent and whether stay fusion generates the readily retrievable pool. Further study is needed to determine whether close fusion contributes to slow endocytosis at synapses. Rapid endocytosis in endocrine cells and neurons is hypothesized to be caused by KR [8] , [19] , [47] , rapid classical endocytosis [46] , [48] or bulk endocytosis [42] , [49] . Which mechanism mediates rapid endocytosis remains unresolved, because each endocytic mode’s contribution had not been reconstructed for comparison with whole-cell endocytosis. Providing such comparison for the first time, we found that close fusion (three close modes), which includes bulk endocytosis (mediated by Ω-enlarge-close), underlies rapid endocytosis ( Fig. 8d , group 1). The three close modes provide a mechanism to regulate vesicle size. Hence, they may contribute to or cause vesicle size variation observed within a cell and among different cells [50] , [51] . Since vesicle size is proportional to quantal size [50] , [51] , regulation of three close modes may in turn modulate quantal size, which defines exocytosis strength, such as increased vesicle size and synaptic strength observed after animal activity [52] . Previous studies suggest that low calcium concentration triggers rapid KR [17] , [18] , which predicts rapid whole-cell endocytosis when calcium influx is reduced or buffered. In contrast, reducing or buffering calcium influx abolishes endocytosis in chromaffin cells and neurons [20] , [22] , [23] , [24] , [53] , [54] . The present work may explain this discrepancy, because in studies suggesting that KR is triggered by low calcium, an indirectly detected Ω-profile, but not pore closure is interpreted as KR [17] , [18] . Such an interpretation is analogous to low calcium-facilitated stay modes reported here ( Fig. 9 ). We found that strong calcium influx triggers close fusion to mediate whole-cell endocytosis, consistent with the finding that calcium influx triggers whole-cell endocytosis ( Figs 8 , 9 ) [20] , [21] , [22] , [23] , [24] , [53] , [54] . Our finding that strong calcium influx triggers close fusion is apparently consistent with results showing that KR is dominant at 90 mM extracellular calcium [14] . However, increasing extracellular calcium (50 mM) decreases ICa during depolarization [15] , implying that prolonged extracellular, but not intracellular calcium increase facilitates KR. Consistent with this implication, prolonged intracellular calcium increase does not promote KR [55] . Taken together, we conclude that strong calcium influx induced by transient depolarization triggers close fusion. Rapid KR (within seconds) is proposed as a simple reversal of fusion pore opening without dynamin involvement, whereas cavicapure (slow KR) may require dynamin [4] , [56] , [57] . The present work provides experimental data showing that not only slow, but also rapid fusion pore closure is mediated by dynamin ( Fig. 9d ). Our finding that close fusion is a dominant endocytic mechanism seems in contrast to the infrequent KR observed in cell-attached recordings. This difference is likely due to different definitions and recording conditions. In cell-attached recordings, KR is detected as equal sized capacitance up- and down-steps that occur within 2 s [7] , [35] , [37] , [58] , [59] , which would exclude Ω-shrink-close, Ω-enlarge-close and Ω-close that closes after 2 s. Furthermore, close modes were triggered by strong calcium influx during transient depolarization ( Fig. 8 ), whereas KR in cell-attached recordings is often detected at rest or with high potassium depoarization [13] , [14] , [35] , [37] , [59] , which does not promote close fusion. How the granule dense core copes with structural changes during Ω-exo–endocytosis is unknown. It might be squeezed out or dissolved first and then released during Ω-shrink [60] , [61] , but might stay as observed in pituitary lactotrophs [61] during stay or close fusion. In summary, the Ω-exo–endocytosis model may explain most live-cell data previously interpreted with FC/KR model. It may apply to large vesicles in many other cell types, such as pancreatic cells, adipocytes, blood cells, glial cells and neurons that secret dopamine, peptides and hormones [62] . Whether it applies to small synaptic vesicles deserves consideration, because neuroendocrine chromaffin cells and nerve terminals are similar in many aspects that were traditionally interpreted with classical exo– and endocytosis models, such as capacitance upsteps and flickers, rapid and slow content release, calcium-triggered rapid and slow endocytosis, bulk endocytosis and proteins involved in exo– and endocytosis [1] , [4] , [5] , [10] , [11] , [20] , [23] , [24] , [63] . Vesicle fusion has been imaged by many techniques, including TIRF [31] or polarized TIRF imaging [64] , two-photon imaging with extracellular dye that our technique is based on [25] , and interference reflection microscopy [42] . Using confocal and STED microscopy, we achieved the highest spatial and temporal resolution currently available, ~90 nm/5–15 ms. We detected pore closure by differential excitation of two dyes at a temporal resolution (~0.3 s) much faster than other imaging methods [31] . Without relying on protein overexpression, our method is much more efficient in capturing vesicle fusion ( Fig. 1e,f ). Our imaging method opens the door for studying the mechanisms that generate and regulate the Ω-profile, or more generally, membrane curvature. Primary bovine chromaffin cell culture We prepared primary chromaffin cell culture as described previously [65] . In brief, fresh adult (21–27 months old) bovine adrenal glands (local abattoir), were immersed in pre-chilled 1 × Lock’s buffer on ice containing: NaCl, 145 mM; KCl, 5.4 mM; Na 2 HPO4, 2.2 mM; NaH 2 PO4, 0.9 mM; glucose, 5.6 mM; HEPES, 10 mM; pH 7.3 adjusted with NaOH. Glands were perfused with 1 × Lock’s buffer, then infused with Lock's buffer containing collagenase P (1.5 mg ml −1 , Roche), trypsin inhibitor (0.325 mg ml −1 , Sigma) and bovine serum albumin (5 mg ml −1 , Sigma) and incubated at 37 ° C for 20 min. The digested medulla was minced in Lock’s buffer and filtered through a nylon mesh. The filtrate was centrifuged (39 g , 4 min), re-suspended in Lock’s buffer and re-centrifuged until the supernatant was clear. Final cell pellet was re-suspended in pre-warmed DMEM low-glucose medium (Gibco) supplemented with 10% fetal bovine serum (Gibco) and plated onto poly- L -lysine (0.005% w/v, Sigma) and laminin (4 μg ml −1 , Sigma)-coated glass coverslips. The cells were incubated at 37 ° C with 8% CO 2 and used within 1 week. Before plating, some cells were transfected by electroporation (2 μg plasmid DNA containing NPY-EGFP or VAMP2-EGFP) using Basic Neuron Nucleofector Kit (Lonza, Program O-005). Electrophysiology At room temperature (22–24 °C), whole-cell voltage clamp and capacitance recordings were performed with an EPC-10 amplifier together with the software lock-in amplifier (PULSE, HEKA, Lambrecht, Germany) [23] , [66] . The holding potential was –80 mV. The frequency of the sinusoidal stimulus was 1,000–1,500 Hz with a peak-to-peak voltage ≤50 mV. The bath solution contained 125 mM NaCl, 10 mM glucose, 10 mM HEPES, 5 mM CaCl 2 , 1 mM MgCl 2 , 4.5 mM KCl, 0.001 mM TTX and 20 mM TEA, pH 7.3 adjusted with NaOH. The pipette (3–6 MΩ) solution contained 130 mM Cs-glutamate, 0.5 mM Cs-EGTA, 12 mM NaCl, 30 mM HEPES, 1 mM MgCl 2 , 2 mM ATP and 0.5 mM GTP, pH 7.2 adjusted with CsOH. These solutions pharmacologically isolated calcium currents. Imaging With an inverted confocal microscope (TCS SP5II, Leica, Germany, 100 × oil objective, numerical aperture: 1.4), A647 (30 μM in bath, Invitrogen) and A488 (30–60 μM in bath, Invitrogen) were excited by a HeNe laser at 633 nm (maximum power: 20 mW) and an Argon laser at 488 nm (maximum power: 25 mW), respectively. Unless mentioned otherwise, the 633 nm laser was set at 60% of the maximum power, whereas 488 nm laser was set at 1.5–2%. A647 fluorescence was collected with a photomultiplier at 643–700 nm, whereas A488, with a GaAsP hybrid detection system at 498–580 nm. The quantum efficiency of the hybrid detection system is two times higher than the photomultiplier, which improved the signal-to-noise ratio for A488 imaging. Both excitation and fluorescence collection were done simultaneously. The inverted STED microscope has a resolution of 80 nm (TCS STED, Leica, Germany), which (~80–90 nm) was confirmed with fluorescent bead measurements. A488 (60 μM) was excited with an Argon laser at 488 nm at 20% of the maximum power (maximum power: 25 mW), and depleted with a continuous wave fiber laser at 592 nm using the maximum power (1.5 W). The fluorescence was acquired by GaAsP hybrid detection system at 498–580 nm. At 20% of the maximum power, 488 nm laser caused A488 bleaching after pore closure with a time course similar to that of A647 under the confocal setting. Confocal or STED imaging area was ~70–160 μm 2 . Images were collected every 5–15 ms at 50–70 nm per pixel at the confocal/A647/A488 setting, every 26 ms at 40 nm per pixel at the STED/cell-bottom setting and every 36 ms at 40 nm per pixel at the STED/cell-centre setting. For imaging at STED/cell-centre setting, we chose a focal plane that showed a clear edge between the solution and the cytosolic compartment of the cell, an indication that the cell membrane was approximately in parallel with the microscope’s z axis. More specifically, at such a focal plane, the distance that covered 20–80% fluorescence changes between the solution and the cytosolic compartment was less than 300 nm, beyond which the cell was not used. Furthermore, to clearly resolve the Ω-profile or the FC profile, we only analysed fluorescent spots with an initial W H more than 350 nm. This selection avoided challenging our limited spatial resolution (~90 nm) when a small spot shrank until undetectable. TIRF imaging (Olympus FV1000) was taken every 100–200 ms with a 60 × oil immersion objective (NA: 1.45) and an EMCCD camera (Hamamatsu Photonics). Alexa 555 in the bath solution was excited by a HeNe laser at 543 nm. Fluorescence measurements and presentations Images were analysed using ImageJ. The fluorescence intensity ( F 647 , F 488 , F STED ) from an area covering the fluorescence spot was measured at every image frame. For images shown in figures and movies, 2–4 frames were averaged at the confocal/A647/A488 setting, 2–3 frames were averaged at STED/cell-bottom setting and 2–8 frames were averaged at STED/cell-centre setting. The averaging improved signals and usually did not sacrifice the time resolution, because most changes were much slower than the time needed for averaging ( Figs 3 , 4 , 5 , 6 ). However, a fraction of ‘shrink’ fusion (Ω-shrink, Ω-shrink-stay, Ω-shrink-close) may take only 50–200 ms during the shrinking phase, in which we used 1–2 frames for averaging. W H was measured from intensity profiles of 1–4 lines (for example, Fig. 2a,b ) across the spot centre at 45° or 90° apart. At STED/cell-centre setting, W H was measured from line profiles approximately in parallel with the cell membrane ( Figs 3c , 4b , 5c,f and 6d ). For line profiles, we normalized the peak fluorescence to 1. For F 647 , F 488 and F STED , the value before the spot appeared was normalized to 1. Identifying fusion modes with a single dye When A647 (strong excitation) and EGFP were imaged ( Fig. 10 ), most fusion modes except Ω-shrink and Ω-close, could be readily distinguished from F 647 change alone, as shown in Figs 3 , 4 , 5 , 6 . Although F 647 decayed in both Ω-shrink and Ω-close fusion, the decay τ for Ω-shrink (1.09±0.11 s, n =115 spots, Supplementary Fig. 13a ) was much faster than that of Ω-close (2.9±0.1 s, n =210 spots, Supplementary Fig. 13b ). Since the decay, τ distribution for Ω-shrink overlapped little with that of Ω-close ( Supplementary Fig. 13c ), we classified spots with a decay τ <1.7 s as Ω-shrink. This criterion excluded Ω-close, because the decay τ for all Ω-close events was >1.7 s ( Supplementary Fig. 13 ). Spots with a decay τ >2 s were classified as Ω-close, in which 8% could be due to Ω-shrink owing to the overlap distribution of the decay τ ( Supplementary Fig. 13c ). Such a small error should not significantly affect our main conclusion. With a single dye (A488, strong excitation) in STED imaging, we identified the fusion modes based on changes in F STED and W H similar to confocal imaging. STED imaging was more sensitive in detecting the W H change, making it easier to distinguish between Ω-shrink and Ω-close. Exo– and endocytosis reconstruction In confocal/A647/A488 experiments, we labelled each spot at the spot onset as an upstep with an amplitude of 1, and a downstep only for three ‘close’ modes at the pore closure time, that is, the onset of A647 bleaching while A488 remained unchanged ( Fig. 8a ). The downstep amplitude was corrected for Ω-shrink-close and Ω-enlarge-close by raising the relative fluorescence changes during the ‘shrink or ‘enlarge’ phase to a power of 2/3, which was approximately proportional to the granule surface area or capacitance. This correction was based on our observation that the fluorescence change was approximately proportional to the W H change raised to a power of 3. Here we did not consider granule size differences for each fusion mode, because the mean spot W H at the fusion onset was similar for seven fusion modes. Measuring the pore closure time For close modes, the onset of the F 647 decay when F 488 remained unchanged was taken as pore closure time. The F 647 decay time constant was 2.9±0.1 s ( n =210), meaning that at 0.3 s, F 647 decays by 10%, which could be well resolved (for example, arrows in Figs 3d–f , 4c and 5d–f ). Thus, our time resolution for pore closure was 0.3 s. If pore closure was less than our resolution, we assigned an arbitrary value of 0.3 s. Data selection for analysis The data within the first 2 min after whole-cell break-in were used to avoid whole-cell endocytosis rundown (see also Fig. 8f ) [21] . Cells showing prominent endocytosis overshoot were discarded, because we focused on determining whether ‘close’ modes are responsible for compensatory endocytosis, and the overshoot often curtailed the capacitance increase to a negative value, making it difficult to compare whole-cell exo–endo with reconstructed exo–endocytosis. Statistics The statistical test used is t- test or paired t- test. The data were expressed as mean±s.e.m. How to cite this article : Chiang, H.-C. et al. Post-fusion structural changes and their roles in exocytosis and endocytosis of dense-core vesicles. Nat. Commun. 5:3356 doi: 10.1038/ncomms4356 (2014).